Heterogeneity of genomic evolution and mutational profiles in multiple myeloma Multiple myeloma is an incurable plasma cell malignancy with a complex and incompletely understood molecular pathogenesis. Here we use whole-exome sequencing, copy-number profiling and cytogenetics to analyse 84 myeloma samples. Most cases have a complex subclonal structure and show clusters of subclonal variants, including subclonal driver mutations. Serial sampling reveals diverse patterns of clonal evolution, including linear evolution, differential clonal response and branching evolution. Diverse processes contribute to the mutational repertoire, including kataegis and somatic hypermutation, and their relative contribution changes over time. We find heterogeneity of mutational spectrum across samples, with few recurrent genes. We identify new candidate genes, including truncations of SP140 , LTB, ROBO1 and clustered missense mutations in EGR1 . The myeloma genome is heterogeneous across the cohort, and exhibits diversity in clonal admixture and in dynamics of evolution, which may impact prognostic stratification, therapeutic approaches and assessment of disease response to treatment. Multiple myeloma (MM) is a malignant monoclonal plasma cell disorder whose pathogenesis is only partially understood. MM is classically subdivided into subtypes with rearrangements involving the immunoglobulin heavy ( IGH ) locus and a hyperdiploid subtype, which harbours multiple trisomies [1] . These chromosomal abnormalities are, however, insufficient for malignant transformation, as they are also observed in monoclonal gammopathy of unknown significance, a premalignant syndrome that precedes virtually every MM case [2] , [3] . MM undergoes a multistep transformation process and its genetic landscape changes over time due to additional events such as somatic mutations, epigenetic and chromosomal copy-number changes driving its progression from monoclonal gammopathy of unknown significance to symptomatic MM and ultimately to aggressive extramedullary disease in some patients [4] . Sequencing efforts in relatively small cohorts of MM samples have already been undertaken, suggesting that MM show a heterogeneous subclonal structure at diagnosis and only few recurrent mutated genes of likely pathogenetic significance, including KRAS , NRAS , TP53 , BRAF and FAM46C [5] , [6] , [7] , [8] . Interestingly, single nucleotide polymorphism (SNP) arrays on serial samples showed that molecular events necessary for MM progression are not attained in a linear fashion but rather through branching, nonlinear pathways [9] , [10] , a pattern typical of a complex ecosystem of clones competing for evolution. The quantitative nature of next generation sequencing (NGS) data allows for higher resolution of the subclonal architecture of cancers [11] and its monitoring over time with implication for prognostic stratification, tumour monitoring and emergence of chemoresistance [12] , [13] . Nevertheless, initial reports of genomic evolution in MM using NGS were conducted again on small cohorts [6] , [8] , thus limiting their relevance to the broadly heterogeneous spectrum of myeloma samples. Importantly, NGS data can also be used to decipher mutational signatures, a combination of mutated nucleotides in a specific context that can inform about mutational processes operative in each cancer and thus offer a mechanistic explanation for the mutations found in the sample [14] . Recent reports suggested that different processes are operative in MM [15] , [16] , [17] , but their relative representation in each sample, the dynamics of their contribution over time and their relation to clinical features are unknown. Here we show the largest cohort to date of MM patients where we combine cytogenetic, copy number and whole-exome-sequencing analysis. We show that most patients have a complex subclonal structure at diagnosis, which evolves further after treatment in the majority of them. We identify mutational processes leading to the generation of MM heterogeneous mutational repertoire, and how they dynamically evolve over time. We describe new candidate driver gene mutations that could inform about disease pathogenesis and prognosis. Landscape of genetic alterations in MM We analysed 84 samples from 67 patients with MM using exome sequencing, high-resolution copy-number arrays and cytogenetics ( Supplementary Tables S1 and S2 ). For 52 patients, one sample was available (pretreatment in 51 cases). 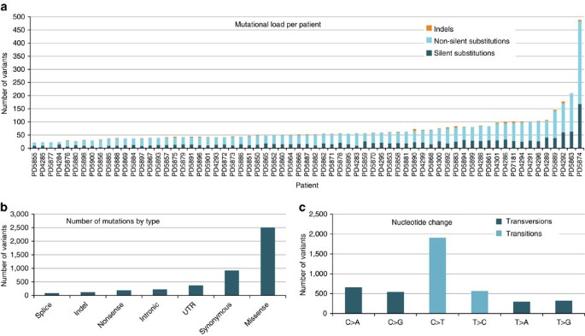Figure 1: Sequencing metrics of the study. (a) Total number of validated somatic variants for each patient in the cohort. (b) Breakdown of variants by type. (c) Breakdown of variants by nucleotide change. Transitions (C>T, T>C) are in light blue, transversions (C>A, C>G, T>A, T>G) in dark blue. We collected serial samples in 15 patients, starting at disease progression or relapse post treatment in 14 of them, with later time points always collected at relapse/progression after further lines of treatment ( Table 1 ). The median interval between samples was 299 days (range 77–618, Supplementary Table S1 ). Table 1 Disease status at the time of sampling. Full size table Exome sequencing, performed at a total average depth of 236 × ( Supplementary Table S3 ), allowed us to identify and validate 4,417 variants (range 21–488, median 52 per patient) ( Fig. 1a , Supplementary Data 1 ). Non-silent coding variants (that is, missense, nonsense, indel, splice) were enriched over silent ones (that is, synonymous, intronic, untranslated region) ( Fig. 1b ). Ranking by mutation type showed an excess of C>T transitions ( Fig. 1c ). We identified 183 homozygous deletions totalling 35.4 Mb ( Supplementary Data 2 ). Figure 1: Sequencing metrics of the study. ( a ) Total number of validated somatic variants for each patient in the cohort. ( b ) Breakdown of variants by type. ( c ) Breakdown of variants by nucleotide change. Transitions (C>T, T>C) are in light blue, transversions (C>A, C>G, T>A, T>G) in dark blue. Full size image From copy-number data, 40/67 patients harboured a hyperdiploid karyotype ( Supplementary Table S2 ). Fluorescence in situ hybridization (FISH) analysis showed 15/67 patients were positive for IGH rearrangements: 6/67 for t(4;14), with increased expression of FGFR3 and MM SET domain; 7/67 for t(11;14), with consequent upregulation of cyclin D1 ; and 2/67 for t(14;16), involving C-maf . Two hyperdiploid samples also carried a subclonal t(11;14) translocation by FISH ( Supplementary Table S2 ). In 12 patients, FISH on IGH rearrangements other than t(4;14) was not available. Other copy-number alterations such as del(1p), (+1q), del(12p), del(13), del(14q), del(16q), del(17p) were found in both hyperdiploid and IGH rearranged cases. The combination of whole-exome sequencing, FISH and copy-number analysis provided an integrated snapshot of the complexity of alterations affecting the myeloma coding genome. Overall, the detection of such a large burden of somatic variants and copy-number alterations, with high variability across the 67 individuals studied, indicates that the genetic landscape of myeloma is remarkably heterogeneous and that largely distinct sets of chromosomal rearrangements and gene mutations are present in individual patients. Modelling clonal and subclonal mutation clusters Cancer evolves through a Darwinian process of clonal expansion, and the population of cancer cells represents an admixture of competing subclones. We explored the clonal structure of our cohort using SNP arrays and whole-exome sequencing data to identify subclonal copy-number changes, simultaneously estimating and adjusting for tumour ploidy and normal cell contamination. A number of cases showed subclonal gains or losses of large-scale genomic regions (examples shown in Supplementary Fig. S1A ). A similar analysis was carried out for point mutations by calculating the 95% confidence interval for the fraction of tumour cells carrying each mutation (again adjusting for the percentage of contaminating normal cells of the sample and the copy number of the locus). Each mutation was classified as clonal (that is, present in all tumour cells) if the upper bound of the 95% confidence interval included 1, and subclonal otherwise. We plotted, for each patient, the absolute number and proportion of clonal and subclonal variants and showed that almost every patient carries variants present in a fraction of tumour cells, implying ongoing tumour evolution at the time of sampling ( Fig. 2a ). We then clustered the fraction of tumour cells carrying each mutation using a Bayesian Dirichlet process, to reflect the clonal composition of the tumour. We showed that all patients carry a cluster of variants that are clonal (that is, at 1.0 on the x axis in Fig. 2b–d , Supplementary Fig. S1B ). Rarely, patients had only few subclonal variants and no significant clustering at the subclonal level ( Fig. 2b ), whereas most patients showed a major cluster of clonal mutations and one or more clusters of subclonal variants ( Fig. 2c , Supplementary Fig. S1B ). Interestingly, few patients had many more subclonal mutations than clonal, in several clusters ( Fig. 2d ), indicating a complex dynamic of tumour evolution from the most recent common ancestor—the most recent tumor cell that has the full complement of somatic mutations found in all tumour cells—through acquisition of new variants in different subclones. 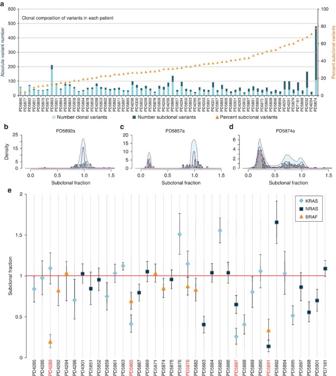Figure 2: Modelling clonal and subclonal mutation clusters. (a) Stacked bar chart showing the number of clonal mutations (present in all tumour cells, light blue) and subclonal mutations (dark blue) in each patient. Also shown is the percentage of subclonal variants (orange triangles). For patients with multiple samples, the fraction of tumour cells used was derived from the earliest sample where the mutation was found. (b–d) Statistical modelling by a Bayesian Dirichlet process of the distribution of clonal and subclonal mutations for three patients for which only one sample was available. For each plot, the faction of tumour cells carrying the variant is represented on thexaxis (1=100% of tumour cells), and the probability density (on an arbitrary scale) on theyaxis. Grey bars represent the histogram of mutations, with the fitted distribution as a dark purple line. The 95% posterior confidence intervals for the fitted distribution are represented by a pale blue area. (b) Patient showing a vast majority of clonal variants; (c) patient with a dominant set of clonal mutations and a minor subclone; (d) patient showing a dominant set of subclonal mutations, at two different proportions. (e) Adjusted fraction of tumour cells carrying KRAS, NRAS and BRAF substitutions found in the study. Error bars represent 95% confidence intervals, accounting for chromosomal copy number of the locus, percentage contaminating normal cells and depth of coverage. (Note that patient PD5883, carrying aBRAFindel, was not included in this panel due to the inaccurate estimation of the allelic fraction of indels). All mutations whose confidence interval includes 1 (red line) are considered to be present in all tumour cells with 95% confidence. Driver mutations can be found at the clonal or subclonal level, and sometimes coexist in the same patient (Patient IDs in red). For patients with multiple samples, the fraction of tumour cells used was derived from the earliest sample where the mutation was found. In three patients (PD5876, PD5885, PD5892), a fraction of ~1.5 was assigned, likely due to focal subclonal gains of the variant locus that went undetected by our algorithms, so that the estimated fraction of tumour cells was not adjusted. Figure 2: Modelling clonal and subclonal mutation clusters. ( a ) Stacked bar chart showing the number of clonal mutations (present in all tumour cells, light blue) and subclonal mutations (dark blue) in each patient. Also shown is the percentage of subclonal variants (orange triangles). For patients with multiple samples, the fraction of tumour cells used was derived from the earliest sample where the mutation was found. ( b – d ) Statistical modelling by a Bayesian Dirichlet process of the distribution of clonal and subclonal mutations for three patients for which only one sample was available. For each plot, the faction of tumour cells carrying the variant is represented on the x axis (1=100% of tumour cells), and the probability density (on an arbitrary scale) on the y axis. Grey bars represent the histogram of mutations, with the fitted distribution as a dark purple line. The 95% posterior confidence intervals for the fitted distribution are represented by a pale blue area. ( b ) Patient showing a vast majority of clonal variants; ( c ) patient with a dominant set of clonal mutations and a minor subclone; ( d ) patient showing a dominant set of subclonal mutations, at two different proportions. ( e ) Adjusted fraction of tumour cells carrying KRAS, NRAS and BRAF substitutions found in the study. Error bars represent 95% confidence intervals, accounting for chromosomal copy number of the locus, percentage contaminating normal cells and depth of coverage. (Note that patient PD5883, carrying a BRAF indel, was not included in this panel due to the inaccurate estimation of the allelic fraction of indels). All mutations whose confidence interval includes 1 (red line) are considered to be present in all tumour cells with 95% confidence. Driver mutations can be found at the clonal or subclonal level, and sometimes coexist in the same patient (Patient IDs in red). For patients with multiple samples, the fraction of tumour cells used was derived from the earliest sample where the mutation was found. In three patients (PD5876, PD5885, PD5892), a fraction of ~1.5 was assigned, likely due to focal subclonal gains of the variant locus that went undetected by our algorithms, so that the estimated fraction of tumour cells was not adjusted. Full size image We next turned our attention to substitutions in known driver genes in myeloma [5] , [6] , [7] . Interestingly, for each of the known driver genes in myeloma ( KRAS, NRAS, BRAF ), we found both patients in whom the mutations were clonal and patients in whom they were subclonal ( Fig. 2e ). Therefore, even variants with known driver potential can be acquired late in myeloma evolution, implying striking variability across patients as to which are early molecular events and which arise later during tumour progression. Another layer of complexity arose in 5/67 samples that surprisingly showed overlap of two or more driver substitutions in KRAS, NRAS or BRAF ( Fig. 2e , patient IDs in red). In PD5878, it can be concluded that KRAS and BRAF both coexisted in the main clone of the tumour, and were therefore both present in all tumour cells. In PD4289, KRAS was present in all tumour cells, while a subclone of cells containing a BRAF mutation evolved later. In other cases, both variants were present at the subclonal level, making it impossible to resolve whether they belong to the same or different clones. If they were in different clones, this would be suggestive of convergent evolution, that is, two different subclones independently acquiring mutations activating the same pathway, as reported in ALL [18] , pancreatic cancer [19] and renal cancer [20] . Clonal evolution We next analysed cases with serial samples. Through analysis of the copy-number patterns, we could track clonal evolution in large-scale genomic aberrations over time ( Fig. 3a–d ). We also clustered point mutations based on clonality again using a Bayesian Dirichlet process, extended into two dimensions to give insights of the changes in the clonal composition of each tumour over time. We plotted the fraction of tumour cells harbouring each variant on the x axis for the ‘early’ sample, and on the y axis for the ‘late’ sample ( Fig. 3ai–di ; Supplementary Fig. S2A ). We observed four major patterns in these paired samples, instructive of genomic evolution over time and possibly across sampling sites [21] . 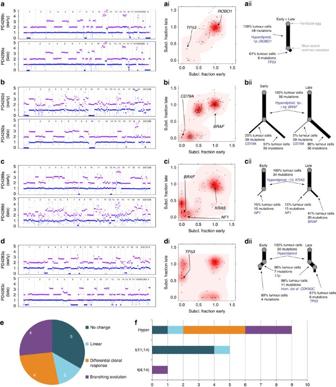Figure 3: Clonal evolution. (a–d) Chromosomal copy-number plots for the early and late sample; in each plot, purple=total copy number, blue=copy number of the minor allele. (ai–di) Two-dimensional density plots showing the clustering of the fraction of tumour cells carrying each mutation (black dots) at each time point; increasing intensity of red indicates the location of a high posterior probability of a cluster. (aii–dii) Phylograms representing the clonal composition of the tumour at each timepoint, where the length of each branch is proportional to the size of the clone (that is, the number of variants), and the width to its clonality (that is, the proportion of tumour cells bearing each variant). Grey circles represent the nodes of the phylograms, that is, the point at which a separate group of cells diverges in evolution from the parental clone. The distance between nodes relates to the evolution time from the fertilized egg down the trunk of the phylograms (that is, the main clone of the tumour), through the most recent common ancestor to the branches of the phylogram (that is, the different subclones of the tumour arisen later in evolution). For each branch, the number and average clonality of the variants has been annotated (black text), along with notable copy-number changes and mutations (dark blue text). (e) Pie chart breakdown of the proportional representation of the different kinds of clonal evolution observed in the cohort. (f) Histograms showing the number of cases and type of clonal evolution for each karyotypic subgroup. Figure 3: Clonal evolution. ( a – d ) Chromosomal copy-number plots for the early and late sample; in each plot, purple=total copy number, blue=copy number of the minor allele. ( a i– d i) Two-dimensional density plots showing the clustering of the fraction of tumour cells carrying each mutation (black dots) at each time point; increasing intensity of red indicates the location of a high posterior probability of a cluster. ( a ii– d ii) Phylograms representing the clonal composition of the tumour at each timepoint, where the length of each branch is proportional to the size of the clone (that is, the number of variants), and the width to its clonality (that is, the proportion of tumour cells bearing each variant). Grey circles represent the nodes of the phylograms, that is, the point at which a separate group of cells diverges in evolution from the parental clone. The distance between nodes relates to the evolution time from the fertilized egg down the trunk of the phylograms (that is, the main clone of the tumour), through the most recent common ancestor to the branches of the phylogram (that is, the different subclones of the tumour arisen later in evolution). For each branch, the number and average clonality of the variants has been annotated (black text), along with notable copy-number changes and mutations (dark blue text). ( e ) Pie chart breakdown of the proportional representation of the different kinds of clonal evolution observed in the cohort. ( f ) Histograms showing the number of cases and type of clonal evolution for each karyotypic subgroup. Full size image In the first pattern we observed, in 5/15 patients, the various clonal and subclonal clusters were found on the leading diagonal of the plots ( Fig. 3ai ) suggesting there was no change in either the mutational profile or the clonal and subclonal composition between the two time points ( Fig. 3aii ). This is rather remarkable, given that these five patients were all treated between the early and late samples, and indeed some had a substantial response as measured by paraprotein levels ( Supplementary Table S1 ). The lack of change in mutational composition suggests that various subclones repopulating the myeloma at relapse were equivalently affected (or unaffected) by treatment. Second, we observed ‘differential clonal response’ in the tumour, in which each subclone was identified at the two time points, but their relative proportions changed over time ( Fig. 3bi,ii ). These changes might reflect random drift of subclones over time, differential response among subclones to chemotherapy or clonal expansion due to selective advantage of one subclone over the others. This pattern was found in 4/15 patients. Interestingly in PD4292, for which three samples were available, we observed differential clonal response in ‘early’ versus ‘late’ and ‘late versus later’ samples. Nevertheless, the drift of subclones at the two intervals was in opposite direction, so that there was actually no change between the first and third sample ( Supplementary Fig. S2A ). This illustrates how different subclones can show alternating dominance over time, likely in this case influenced by treatment. Third, we observed linear evolution in 2/15 patients, in which a new subclone emerged in the late sample that was not evident despite the deep sequencing in the earlier sample ( Fig 3ci,ii ). Fourth, we found evidence of branching evolution in 4/15 patients ( Fig. 3di,ii ). Here, in the time between the early and late time points, one or more new clones have emerged, whereas others have declined in frequency or disappeared. We found striking concordance between point mutations and copy-number changes ( Fig. 3a–d , Supplementary Fig. S2B ), so that karyotypic changes of prognostic value were only observed between paired samples showing linear or branching evolution ( P =0.0002, Fisher exact test). This concordance suggests that the mutational processes acting at the level of point mutations and at the level of aneuploidy in myeloma are broadly in concert over time and across subclones. Surprisingly, the pattern of genomic evolution could not be predicted by response to treatment, interval between sampling or treatment type. We noted that 4/5 cases with the t(11;14) translocation showed no change, as compared with only 1/9 in the hyperdiploid group ( P -value from Fisher test =0.023, Fig. 3f ), suggesting that cytogenetic subtypes can show different evolution in response to treatment. Cases showing either branching evolution or differential clonal response highlight how current anti-myeloma treatment can have a differential effect across subclones, suppressing some and leaving others untouched. While this could have implications for the choice of treatment modalities and for the definition of disease response, larger sample sizes would be important to explore these points in more detail. In our cohort of 15 patients with serial samples, we found no differences in the survival based on the type of genomic evolution shown at relapse. Interestingly, the two most distinct examples of branching evolution (PD4283 and PD4301) came from patients where the late samples represented an extramedullary relapse of myeloma (secondary plasma cell leukaemia and malignant ascites, respectively). Not surprisingly, acquired variants in the late samples included mutations in genes with known oncogenic potential in MM. In the plasma cell leukemia sample, we found a TP53 mutation and a homozygous deletion of CDKN2C ( Fig. 3di,ii ). In the ascites relapse, there were new clonal mutations in NRAS , NFKBIA and FAM46C ( Supplementary Fig. S2 ). Finally, we looked at mutations in five known driver myeloma genes ( KRAS , NRAS , TP53 , BRAF , FAM46C ) across all patients with serial samples, and identified 12 non-silent variants. Six out of twelve were clonal at both time points. Of the remaining, 4/6 appeared in the late sample with no evidence in the early sample despite high-sequence coverage, and 2/6 were subclonal at the initial time point and increased their clonal fraction at the later time point, consistent with the expected positive selection for the subclones harbouring them ( Supplementary Fig. S2C ). Different mutational processes active in MM The catalogue of somatic mutations in a cancer is the aggregate outcome of strength and duration of exposure to one or more mutational processes. Each process generates mutations characterized by a specific combination of nucleotide change and nucleotide context, therefore providing a ‘signature’ that can be used for its identification. Because there are six classes of base substitution (that is, C>A, C>T, C>G, T>A, T>C and T>G; all in pyrimidine context) and 16 possible sequence contexts for each, there are 96 possible mutated trinucleotides, whose relative contribution we represented as a heatmap for each case ( Supplementary Fig. S3A ). We then employed a nonnegative matrix factorization (NMF) and model selection approach to extract mutational signatures from all cases [22] . Evaluation of NMF decompositions suggested that at least two biologically distinct mutational signatures were present ( Fig. 4a ). Each signature was characterized by a different profile of the 96 potential trinucleotide mutations and contributed to a different extent to each cancer. The most represented signature, named Signature A ( Fig. 4a ), is a rather generic mutation signature with enrichment of C>T transitions at CpG dinucleotides, an intrinsic mutational process reflecting spontaneous deamination of methylated cytosine to thymine. A similar signature is dominant in myeloid malignancies [23] , [24] , a major contributor to early mutations in breast cancer [11] , [22] and seen at high rates in the germline [25] . Potentially, other signatures operative in MM could be admixed in Signature A, but larger studies will be required to pursue this observation. A second signature, namely C>T, C>G and C>A mutations in a TpC context (Signature B, Fig. 4b ), was the major contributor of mutations in a few samples ( Fig. 4c ). In PD5863 and PD5874, the two patients with the highest overall number of variants ( Fig. 1a ), virtually all of the mutational repertoire could be attributed to Signature B. While mutations attributed to Signature B were generally spread across the exome, in two samples we found clusters of 4–6 cytosine mutations at TpC dinucleotides within an interval of few hundred bp that also showed strand specificity, indicative of a process known as ‘kataegis’ [22] ( Supplementary Fig. S3B , arrows). Both the genome-wide and the clustered variants of this mutational signature were first documented in breast cancer [11] , [22] , [26] , and are hypothesized to result from the aberrant activity of APOBECs, a family of proteins that enzymatically modify single-stranded DNA [27] . While the genome-wide variant of Signature B was recently described in MM [15] , [16] , here we report the first evidence of clusters of kataegis in this disease. 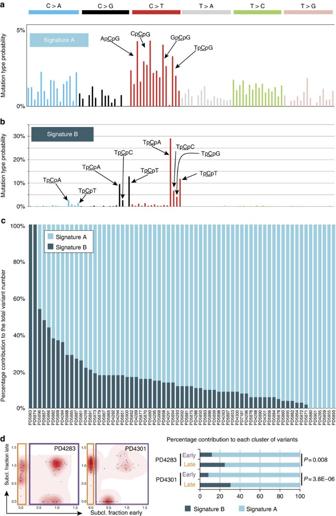Figure 4: Mutational processes operative in multiple myeloma. (a,b) Fraction of contribution of each mutation type at each context for the two mutational signatures identified by NMF analysis. The major components contributing to each signature are highlighted with arrows. (c) Stacked bar chart showing the percentage contribution of the two mutational processes identified by NMF to the total number of variants present in each case. Dark blue bars=Signature B, light blue bars=Signature A. (d) In two examples of branching evolution, PD4283 and PD4301, the percentage contribution of the two mutational processes identified by NMF to the variants present in the early sample (dark purple box) was compared with that of the new variants in the late sample (orange box). A stacked bar chart shows that the contribution from Signature B increases significantly in the ‘late’ variants (χ2test). Dark blue bars=Signature B, light blue bars=Signature A. Figure 4: Mutational processes operative in multiple myeloma. ( a , b ) Fraction of contribution of each mutation type at each context for the two mutational signatures identified by NMF analysis. The major components contributing to each signature are highlighted with arrows. ( c ) Stacked bar chart showing the percentage contribution of the two mutational processes identified by NMF to the total number of variants present in each case. Dark blue bars=Signature B, light blue bars=Signature A. ( d ) In two examples of branching evolution, PD4283 and PD4301, the percentage contribution of the two mutational processes identified by NMF to the variants present in the early sample (dark purple box) was compared with that of the new variants in the late sample (orange box). A stacked bar chart shows that the contribution from Signature B increases significantly in the ‘late’ variants ( χ 2 test). Dark blue bars=Signature B, light blue bars=Signature A. Full size image Kataegis was not the only process leading to regional clustering of mutations in the cohort. We found clusters of mutations in the first exon of CCND1 in two cases ( Supplementary Fig. S3C , arrows), both characterized by the t(11;14) translocation, juxtaposing CCND1 with the IGH locus. Interestingly, selection analysis of the mutations in CCND1 in our cohort revealed that the observed mutations reflected a local mutation rate much higher than the genomic average ( Supplementary Table S4 ). The breakpoints on 11q13 are dispersed over 330 kb centromeric to CCND1 (ref. 28 ), and thus we do not believe that this could arise from the proximity of CCND1 to the site of rearrangement. Rather, the even representation of cytosine and adenine mutations and the high synonymous to non-synonymous ratio suggest CCND1 mutation clusters may result from somatic hypermutation driven by the AID protein [29] , [30] , as previously described for CCND1 itself in mantle cell lymphoma [31] and for BCL2 in follicular lymphomas [32] . We found that CCND1 was significantly enriched for mutations in AID recognition motifs ( Supplementary Fig. S3C ), further reinforcing this hypothesis. Last, we analysed the contribution of each signature, over time or across subclones, in seven patients where the number of variants was high enough to allow a statistical analysis. We observed a significant change in contribution from the two signatures in 5/7 patients. In both cases of extramedullary relapse showing branching evolution, the contribution from Signature B increased significantly at relapse ( Fig. 4d ), and in PD4301d, clustered in a pattern consistent with kataegis ( Supplementary Fig. S3Bi ). Conversely, in the five other samples, we found that the contribution of Signature B could either increase or decrease over time or in different subclones ( Supplementary Fig. S3D ). Overall, the representation of Signature B at relapse was not predictive of the type of genomic evolution shown or of survival. In summary, the MM genome is shaped by several different mutational processes. These are likely to include spontaneous deamination of methylated cytosine, kataegis and somatic hypermutation. The scale of such mutational processes can vary from genome wide to localized clusters of events, and frequently changes over time. Further studies will be required to ascertain whether the relative contribution of different mutational processes can influence clinical outcome or can be influenced by treatment. Recurrently mutated genes in MM We next analysed our data set to identify genes that were mutated with a significant recurrence rate, and could therefore represent novel candidate driver genes in MM. We applied a frequentist likelihood ratio test to highlight genes with increased numbers of non-synonymous substitutions and indels, relative to that expected for the synonymous mutation rate. Through this algorithm, we found seven genes recurrent with a high level of confidence (false discovery rate (FDR)<0.10, asterisks in Fig. 5b ). Mutations of genes involved in the mitogen-activated protein kinase (MAPK) pathway were the most prevalent (37/67 patients). Known KRAS and/or NRAS -activating mutations were present in 32/67 patients. BRAF mutations were present in 10/67 cases. While 9/10 BRAF mutations were previously reported in the literature, only 3/10 were the classic V600E, an atypical feature compared with melanoma or colorectal cancers. Other than these recurrently mutated genes, we found occasional mutations in other genes involved in MAPK signalling, such as NF1 and RASA2 , a negative regulator of RAS signalling [33] . Surprisingly, we again found significant overlap, and two or more mutations activating the MAPK pathway coexisted in 7/67 patients ( Fig. 5b ). 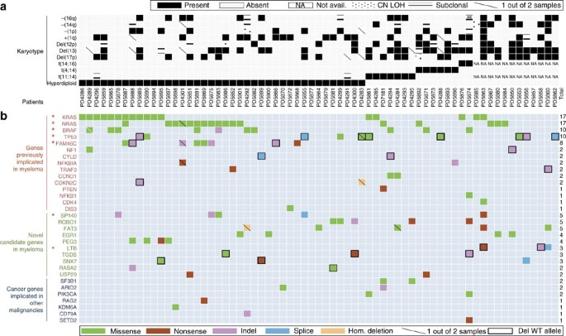Figure 5: Landscape of genetic alterations and recurrently mutated genes in multiple myeloma. Table highlighting relevant genetic alterations and recurrently mutated genes in the study. Patients are represented in columns. (a) Karyotypic features of each patient. (b) Recurrently mutated genes, color coded for missense (green), nonsense (red) and splice-site (blue) substitutions; indels are in light purple and homozygous deletions in ocra. For patients with serial samples, events occurring only in one sample only are highlighted with a diagonal bar. In case of multiple mutations in the same gene in a patient, only one is plotted. In case a mutation is associated with the deletion of the wild-type allele, the gene shows a black contour. For each gene, the number of patients harbouring at least one non-silent mutation is provided in the ‘TOTAL’ column. Asterisks mark genes mutated at a significant recurrence rate in the data set (P-value<0.02 and false discovery rate of <10%). Figure 5: Landscape of genetic alterations and recurrently mutated genes in multiple myeloma. Table highlighting relevant genetic alterations and recurrently mutated genes in the study. Patients are represented in columns. ( a ) Karyotypic features of each patient. ( b ) Recurrently mutated genes, color coded for missense (green), nonsense (red) and splice-site (blue) substitutions; indels are in light purple and homozygous deletions in ocra. For patients with serial samples, events occurring only in one sample only are highlighted with a diagonal bar. In case of multiple mutations in the same gene in a patient, only one is plotted. In case a mutation is associated with the deletion of the wild-type allele, the gene shows a black contour. For each gene, the number of patients harbouring at least one non-silent mutation is provided in the ‘TOTAL’ column. Asterisks mark genes mutated at a significant recurrence rate in the data set ( P -value<0.02 and false discovery rate of <10%). Full size image Thus, MAPK signalling is frequently activated in myeloma and inhibition of this pathway could represent a valid therapeutic target. We therefore examined the sensitivity of nine myeloma cell lines, of which four carried BRAF or RAS mutations, to a panel of BRAF and MEK inhibitors [34] . Among these lines, there were no striking differences in IC50 attributable to genotype, nor any general sensitivity of myeloma lines to these inhibitors compared with other cancers ( Supplementary Fig. S4 ). While the number of lines examined is small, the pattern of response to these inhibitors is similar to colorectal cancers with BRAF mutations, which overcome BRAF inhibition by feedback activation of other proliferative pathways [35] . Another significant gene in our cohort is FAM46C , recently confirmed to be a target of recurrent mutations in myeloma [5] , [7] , [36] . We found eight patients carrying FAM46C mutations, statistically associated with a hyperdiploid karyotype ( P =0.02, Fisher exact test). While in the original reports the pattern of mutations was rather hard to interpret, we find five truncating mutations, two in-frame indels and four missense mutations, three of which clustered in amino acids 138–145 ( Fig. 6 ). In patient PD5868, we identified two truncating mutations, and in PD5891, we found three missense mutations with different clonality. Unless all mutations are in the same allele, this is suggestive of either compound heterozygosity or convergent evolution in separate subclones. Furthermore, patients PD5866 and PD5888 showed a truncating mutation associated with deletion of the remaining wild-type allele ( Fig. 5a,b ). The high rate of inactivating mutations and gene deletions in our data clarifies that FAM46C is a bona fide tumour-suppressor gene in MM [37] . TP53 mutations were found in 10 patients, and were significantly enriched in cases with del(17p) ( P =0.01, Fisher exact test). We also describe additional genes mutated at a significant recurrence rate, and thus novel candidate drivers in MM. SP140 , a lymphoid-restricted homologue of SP100 that encodes a nuclear body protein implicated in antigen response of mature B cells [38] , showed four truncating (2 frameshift, 1 nonsense, 1 splice site) and one missense mutation ( Fig. 6 ). LTB , a type II membrane protein of the TNF family involved in lymphoid development, showed clustered truncating mutations in three samples ( Fig. 6 ), two of which were associated with the loss of the wild-type allele ( Fig. 5b ). LTB heterodimerizes with LTA to generate the ligand for LTBR [39] , which is a positive regulator of the NF-kB pathway, frequently amplified in MM [40] , [41] . This significant frequency of inactivating somatic mutations suggests that SP140 and LTB are novel candidate tumour suppressors in MM. 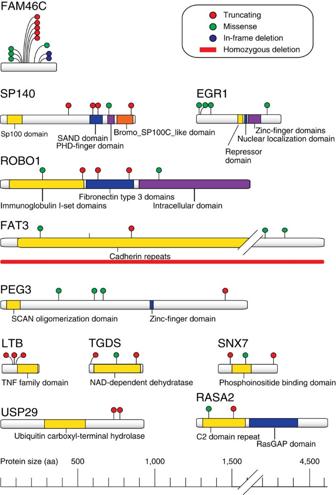Figure 6: Novel gene mutations identified in multiple myeloma. Schematic representation of known or predicted functional domains (from NCBI) of the protein products of the main novel genes identified in the screen, and location of the observed variants, color coded by type: red=truncating variants (nonsense, out-of-frame indels, essential splice-site mutations), green=missense variants, and blue=in-frame indels. FAT3 shows a homozygous deletion spanning the whole locus in a patient and this is shown by a red bar. Figure 6: Novel gene mutations identified in multiple myeloma. Schematic representation of known or predicted functional domains (from NCBI) of the protein products of the main novel genes identified in the screen, and location of the observed variants, color coded by type: red=truncating variants (nonsense, out-of-frame indels, essential splice-site mutations), green=missense variants, and blue=in-frame indels. FAT3 shows a homozygous deletion spanning the whole locus in a patient and this is shown by a red bar. Full size image Using less stringent cutoffs ( P <0.02 and FDR >0.10, see ‘Statistical analysis of recurrently mutated genes’ under Methods) to identify novel genes involved in MM, we highlighted a number of candidates ( Supplementary Table S4 ). ROBO1 , a transmembrane receptor implicated in beta-catenin and MET signalling and recently reported as mutated in pancreatic cancer [42] , was mutated in 5/67 patients. Strikingly, three of these mutations were truncating, consistent with the copy-number loss seen in pancreatic cancer ( Fig. 6 ). The EGR1 gene, which encodes the early growth response one transcription factor, carried four missense mutations ( Fig. 6 ), as well as being mutated in two additional myeloma patients in the literature [5] . FAT3 , a transmembrane protein belonging to the Cadherin superfamily [43] showed a homozygous deletion, one nonsense and three missense mutations ( Fig. 6 ). Looking at genes targeted by both mutations and copy-number variations, we highlighted TGDS , a gene encoding enzyme involved in nucleotide sugars metabolism [44] located in chromosome 13, and SNX7 , a member of the sorting nexin family involved in intracellular trafficking [45] located in 1p21.3. Both genes reside in commonly deleted regions in myeloma, and both showed two truncating and one missense mutations associated with loss of the WT allele ( Fig. 5a,b ). Finally, we found a cluster of mutations involving two neighbouring paternally imprinted genes that share transcriptional regulation [46] in 6/67 patients. PEG3, a gene involved in NF-kB/TNF signalling [47] , and USP29, a poorly characterized deubiquitinating enzyme involved in p53 stabilization [48] , showed a total of three nonsense and three missense mutations, suggesting this locus could be a recurrent target of mutations in MM ( Fig. 6 ). Manual inspection of the gene list allowed the identification of several mutations in other genes previously implicated in lymphoid malignancies, although at a non-significant recurrence rate ( Fig. 5b ). Across our 67 patients, we find a missense variant affecting the ankyrin repeat domain in NFKB1 and two truncating somatic mutations each in NFKBIA , CYLD and TRAF3 . These data confirm that the non-canonical NF-kB pathway is an important target for somatic mutation in MM [41] . We also find somatic mutations in genes involved in B-cell development, such as a nonsense mutation in RAG2 (deleted in ALL) and a frameshift mutation in CD79A (mutated in diffuse large B-cell lymphoma). Rare mutations were also found in other cancer genes, including SF3B1 (three missense mutations in two patients); ARID2 (one frameshift, one missense); PIK3CA (two recurrent missense mutations); PTEN (one nonsense); KDM6A (one homozygous deletion); CDK4 (one missense); CDKN2C (one frameshift, one homozygous deletion); and SETD2 (one nonsense). In four patients, RNA-seq data were available, and we confirmed that most of the known and candidate driver genes in myeloma are expressed in the tumour cells, although at variable levels ( Supplementary Fig. S5A ). In seven additional patients, RNA was available for RT–PCR. We showed that eight out of the 10 mutations we investigated were expressed, suggesting good correlation between DNA mutational status and expression of mutated driver genes ( Supplementary Fig. S5B ). Interestingly, a nonsense mutation in the paternally imprinted gene PEG3 showed a homozygous-mutated peak, confirming hemizygous expression of the mutated allele and predicting loss of function of the locus ( Supplementary Fig. S5B , panel 9). Relapse-free ( Supplementary Fig. S6A–F ) and overall survival data ( Supplementary Fig. S6Ai–Fi ) were available for the 51 patients sampled at diagnosis. We found, as previously reported [1] , that hyperdiploid cases had longer overall survival than those with IGH translocations ( Supplementary Fig. S6Fi ). We found no significant difference in overall and relapse-free survival between cases with mutations in KRAS , NRAS or BRAF compared with those without. Similarly, we found no effect of mutations in FAM46C , EGR1 , LTB or ROBO1 . Presence or absence of a subclonal driver mutation did not influence clinical outcome either. Interestingly, TP53 and SP140 mutations correlated with shorter relapse-free survival, but both had no effect on overall survival ( Supplementary Fig. S6B,D,Bi,Di , respectively). We then looked at the influence of the overall mutational spectrum on survival. We found no difference in patients with higher fraction of mutations generated by Signature B, or higher fraction of subclonal mutations ( Supplementary Fig. S6A,C,Ai,Ci , respectively). Conversely, increased number of variants correlated with a higher risk of relapse and death ( Supplementary Fig. S6E,Ei ). Sample sizes here are clearly limited, and defining the prognostic role of such variables will require considerably larger cohorts. In this study, we report the largest myeloma cohort to date where the coding exome of purified tumour cells was investigated by NGS. The selection of patients in our study was somewhat different to previously published reports, with overrepresentation of advanced disease, hyperdiploid and del(17p) cases and underrepresentation of t(11;14) and t(4:14). This may explain the low frequency of DIS3 mutations (mostly found in IGH rearranged cases so far [5] , [7] ), and higher prevalence of TP53 and FAM46C variants. The depth of sequencing in our study was higher than the one from other reports, and we validated every variant that was reported by the initial whole-exome sequencing. This allowed for the validation of numerous low burden variants, and provided enough resolution to dissect the subclonal structure of the tumours. We confirm previous reports showing subclonal KRAS , NRAS and BRAF mutations in MM [7] that we observe in about a third of patients. This will be relevant in trials of MEK and BRAF inhibitors, as their therapeutic effect should be maximal only in cases where these driver mutations are present in all tumour cells. We show for the first time concurrent BRAF and NRAS or KRAS mutations at diagnosis in the same patient, another finding that has therapeutic implications. BRAF inhibitors can have a paradoxical ERK-activating effect in RAS -mutated cells, therefore inducing secondary tumours driven by oncogenic RAS [49] , [50] . This suggests that there may be paradoxical tumour-enhancing effects of BRAF inhibitors in patients with coexistent BRAF and RAS mutations. Furthermore, the presence of mutations of two genes involved in the MAPK pathway in the same patient raises the possibility that MM shows features of convergent evolution and underscores the relevance of this pathway for MM pathogenesis, but also the challenges to exploit it for therapeutic purposes. Our large cohort allowed for a more comprehensive analysis of recurrently mutated genes in MM compared with previous studies, which resulted in novel findings. We confirm that FAM46C is recurrently inactivated in MM in a pattern typical of a tumour-suppressor gene, and associates with the hyperdiploid subgroup of MM. We describe novel candidate tumour-suppressor genes hit by recurrent inactivating mutations at a significant rate, such as SP140 and LTB . Interestingly, SP140 is expressed to high levels in plasma cells and linked to germline susceptibility to CLL [51] . The germline risk allele is associated with reduced expression of SP140 in lymphocytes [51] , which would be consistent with the observations of truncating mutations here. Furthermore, the increased risk of relapse associated with SP140 mutations in our cohort suggests this gene may have prognostic features in MM. Another recurrently mutated gene, EGR1 , encodes a protein that acts downstream of the JUN pathway, enacting an apoptosis programme in MM cells through downregulation of survivin and upregulation of caspases [52] . Knockdown of EGR1 in myeloma cells enhanced their resistance to bortezomib [52] , and the clustered point mutation of key residues that we observed may have similar effects. We show that the heterogeneous subclonal structure and mutational repertoire of MM samples is generated by at least two mutational processes. The relative contribution of each process changed over time or within subclones in most patients, and the contribution of Signature B increased most markedly in the two patients presenting with extramedullary relapse of MM and showing distinct branching evolution. This suggests that the ability to grow independently of the bone marrow microenvironment is gained through substantial changes in the genome of the neoplastic plasma cells. Nevertheless, we fail to demonstrate a correlation between survival and either the prevalence of a specific mutational signature, or the different levels of subclonal complexity of each tumour. Rather, we show that cases with significantly higher number of mutations had worse relapse-free and overall survival, regardless of how mutations were generated or distributed across subclones. In light of recent data showing that the number of variants in MM correlates with stage of disease [8] , our findings suggest that more advanced disease at diagnosis negatively impacts the clinical outcome. The presence of high variability in genomic architecture across samples highlights the need for therapeutic interventions directed at multiple targets rather than a single genomic anomaly, and underscores the striking success of combination therapies with proteasomal inhibitors and immunomodulatory agents [53] . As we move towards an era of personalized therapy for myeloma and other cancers, we need to build an understanding of the recurrently mutated genes, their effect on drug response and the impact of the admixture of subclones containing specific mutations on initial presentation, therapy and relapse. The well-established practice of serial bone marrow examination to monitor disease status, the complexity of the genomic landscape and the rapidly evolving therapeutic options suggests MM is a powerful testbed for this vision. Sequencing and genomic alignment The study involved the use of human samples, which were collected after written informed consent was obtained. Samples and data were obtained and managed in accordance with the Declaration of Helsinki under protocol 08/H0308/303: somatic molecular genetics of human cancers, Melanoma and Myeloma (Dana Farber Cancer Institute). The same protocol was approved by RES Committee East of England—Cambridge Central. We sequenced the protein-coding exome of 84 tumour samples from 67 patients with MM. DNA was isolated from CD138-positive myeloma cells purified from bone marrow, and constitutional control DNA originated from peripheral blood mononuclear cells. Purity of the CD138+ fraction was assessed by anti-CD138 immunocytochemistry post sorting, and only samples with >90% plasma cells were sequenced. Two ( n =13) or three ( n =2) serial samples were available for 15 patients. Fifteen patients were sampled at disease relapse, including 14 with serial samples, and 52 were sampled before treatment. Karyotype and/or FISH data were available for all patients, and the Affymetrix Genome-Wide Human SNP Array 6.0 (SNP6) was performed in 19/84 samples ( Supplementary Table S1 ). Genomic libraries enriched for protein-coding exons were generated by hybridization to RNA baits from matched tumour and germline DNA samples, using the Agilent SureSelect Human Exon Kit (Agilent, G3362) [54] . The libraries, containing an average insert size of 200–300 bp, were analysed on the Illumina HiSeq2000 sequencing platform. Paired 75 bp sequencing reads were generated using the standard protocol. Paired-end sequencing reads were aligned to the human genome (NCBI build37) using the BWA algorithm [55] . Reads which were unmapped, PCR-derived duplicates or outside the targeted region were excluded from analysis. The remaining uniquely mapping reads provided an average of 75.38% coverage over the targeted exons at a minimum depth of 30 × ( Supplementary Table S2 ). To identify somatically acquired coding point mutations, we used CaVEMan (Cancer Variants through Expectation Maximization) [23] , [54] , an algorithm that uses a naïve Bayesian classifier to estimate the posterior probability of each possible genotype (wild type, germline SNP, somatic mutation) at a given base, accounting for the effects of observables such as base quality (measuring signal-to-noise ratio), read position, sequencing lane and read orientation. CaVEMan is configured to incorporate knowledge of copy number and normal cell contamination in the posterior probability calculations. To call insertions and deletions, we used split-read mapping implemented as a modification of the Pindel algorithm [56] . We include in the search for indels read-pairs in which one or both ends map to the genome, but allow one of the pair to have mismatches, insertions or deletions. Pindel searches for reads where one end is anchored on the genome, and the other end can be mapped with high confidence in two (split) portions, spanning a putative indel. All somatic coding mutations underwent validation regardless of their allelic fraction. For a fraction of the variants (~25%), we used PCR followed by massively parallel pyrosequencing (Roche 454) [26] . For the remainder, new libraries were produced after whole-genome amplification, and variants were validated by hybridization and pull-down with a custom bait set. The allelic fraction of variants in the original whole-exome study (on native DNA) and that of the targeted pull-down validation (on amplified DNA) were combined since they showed a near-perfect correlation ( r =0.89, P =<2.2e−16, Pearson's product-moment correlation), implying that whole-genome amplification did not introduce bias in our data. In serial samples, each variant was validated in all samples from that patient. For variants validated by Roche 454, coverage (~100 × on average) and allelic fraction data came from the original whole-exome study. The sensitivity of our pipeline to detect a given subclonal mutation was previously shown on whole-genome sequencing data to vary, and is especially dependent on coverage across the mutated base and the extent of normal cell contamination [11] . For our study, based on exome data, we sample less of the genome but do so at higher depth. Thus, our sensitivity to detect at least a fraction of the subclonal mutations was high, as evidenced by the fact that we robustly detect and validate mutations down to 5–10% of tumour cells. Copy-number analysis and fraction of mutated cells estimates SNP array hybridization on the Genome-Wide Human SNP Array 6.0 (Affymetrix) platform was performed ( Supplementary Table S1 ) according to the manufacturer protocols [57] for 19 out of 84 samples of the exome screen. For the remaining 65 samples, copy-number data were derived from exome-sequencing data. Copy-number analysis was performed using ASCAT (version 2.2) taking into account non-neoplastic cell infiltration and tumour aneuploidy and resulted in integral allele-specific copy-number profiles for the tumour cells [58] . ASCAT output was compared with karyotype/FISH analysis, where available, showing a highly significant correlation: the P -value reflecting the correlation between ASCAT and FISH analysis for hyperdiploidy, del(13) and del(17p) was <2.2e−16, <2.2e−16 and 3.615e−12, respectively (Fisher exact test). It was previously reported that ASCAT can reliably identify clonal and subclonal copy-number changes in tumours using SNP6 or whole-exome sequencing data [26] , [58] and our data further reinforce this evidence [26] , [59] . Homozygous deletions were called if there were zero copies in the tumour cells. The mutation copy number, n mut , equivalent to the fraction of tumour cells carrying a given substitution multiplied by the number of chromosomal copies of the mutation, n chr , was estimated as previously described [26] , using: where f s is the fraction of mutated reads observed in the sequencing data, and ρ , and are respectively the tumour purity, the locus-specific copy number in the tumour cells and the locus-specific copy number in the normal cells, inferred from ASCAT. The confidence intervals for the mutation copy numbers were generated by bootstrap resampling the wild-type and mutant reads at each mutated locus ( n =10,000) and applying the above formula to the resampled fractions of reads. The mutation copy number reflects the percentage of tumour cells carrying the mutation, and allows comparison across samples with different karyotypes and fraction of contaminating normal cells. Thus, heterozygous mutations occurring at a diploid locus, and mutations occurring at a locus that underwent heterozygous or subclonal deletion of the WT allele are assigned the same mutation copy number. Note that indels were excluded from this analysis because of potential mapping bias that would decrease the confidence in quantifying their allelic fraction. Mutations that are present on multiple copies of a chromosome or chromosome segment as a result of a copy-number aberration will have mutation copy numbers above 1. In order to group mutations by the fraction of cells containing a mutation, the number of chromosomes bearing a mutation, n chr , must be known. For all mutations in amplified regions with major copy number C, the observed number of mutant and wild-type reads was compared against the expected f s values resulting from the mutation being present on 1, 2,…C chromosome copies, assuming a binomial distribution, and n chr was assigned the value of C with the maximum likelihood. The fraction of cells bearing each mutation was then calculated as n mut / n chr . 1D and 2D variant clustering The plots in Fig. 2b–d and Supplementary Fig. S1 were produced using a previously developed Bayesian Dirichlet process to model clusters of clonal and subclonal point mutations, allowing inference of the number of subclones and the fraction of cells within each subclone [11] . Within this model, the number of reads bearing the i th mutation, y i , was drawn from a binomial distribution where N i is the total number of reads at the mutated base and ζ i is the expected fraction of reads that would report a mutation present in 100% of tumour cells at that locus. π I ε(0, 1), the fraction of tumour cells carrying the i th mutation, was modelled as coming from a Dirichlet process DP, with concentration parameter α . We used the stick-breaking representation of the Dirichlet process: where ω h is the weight of the h th mutation cluster, that is, the proportion of all somatic mutations specific to that cluster. For those patients with multiple samples, this model was extended into two dimensions, with the number of mutant reads obtained from a pair of samples obtained at different time points, y i,1 and y i,2 , modelled as independent binomial distributions, each with an independent π drawn with a Dirichlet process from a base distribution U(0,1). for both the one-dimensional and two-dimensional models, Gibbs sampling was used to estimate the posterior distribution of the parameters of interest, implemented in R, version 2.11.1. The Markov chain was run for 10,000 iterations, of which the first 2,000 were discarded. The median of the density was estimated from π h , each weighted by the associated value of ω h , using a univariate or bivariate Gaussian kernel, implemented in the R libraries stats and KernSmooth , respectively. The sensitivity of this approach in detecting clusters of subclonal mutations was previously estimated [11] , and was found to be dependent on coverage, on the fraction of contaminating normal cells and number of mutations within the subclone itself. Mutational processes and signature analysis Signatures of mutational processes were analysed using the Wellcome Trust Sanger Institute mutational signatures framework [14] . Statistical analysis of recurrently mutated genes We used a model-based approach (frequentist likelihood ratio tests) to classify genes based on their observed patterns of recurrent mutation, based on ref. 60 . In this method, the expected number of non-synonymous mutations in a given gene is modelled as a product of the number of vulnerable sites, the mutation rate of each type of substitution and a separate selection coefficient for each gene and each type of non-synonymous substitution. This allows quantifying selection at gene level avoiding the confounding effects of gene length, sequence composition and different rates of each substitution type. We used a likelihood implementation of this model to evaluate whether the frequency of missense, nonsense, splice-site substitutions and indels is higher than expected by chance. Twelve parameters were used to model the 12 possible single nucleotide substitutions and two additional parameters control for the CpG effect on C>T transitions in each strand. Three selection parameters ( w mis , w non and w splice ) quantified selection at missense, nonsense and essential splice-site substitutions, respectively. Maximum likelihood was used to estimate these parameters and likelihood ratio tests were used to test deviations from neutrality ( w mis =1, w non =1 or w splice =1). Since the limited number of mutations per gene prevents the estimation of different rates per gene, mutation rates were assumed constant among genes and only the three selection parameters were allowed to vary, thus reflecting a ratio between the observed and the expected numbers of missense, nonsense, splice-site substitutions and indels per gene. Nevertheless, an additional likelihood ratio test was performed to identify those genes whose number of synonymous mutations significantly deviates from the assumed uniform mutation rate. This analysis identified CCND1 as the only gene with a significantly higher background mutation rate in the data set. For indels, a P -value was obtained for each gene comparing the observed number of indels to the expected number (estimated as the product of the CDS length and the exome wide average indel rate per bp) using a cumulative Poisson distribution. For each gene, the four P -values for indels, missense, nonsense and splice-site mutations were combined using Fisher method. P -values were adjusted for multiple testing using Benjamini–Hochberg FDR. Accession codes: The whole-exome sequencing data have been deposited in the European Genome-phenome Archive (EGA) repository under the accession code kEGAD00001000339 Data from SNP array hybridization on the SNP6.0 platform have been deposited in EGA under the accession code EGAD00010000395. How to cite this article : Bolli, N. et al. Heterogeneity of genomic evolution and mutational profiles in multiple myeloma. Nat. Commun. 5:2997 doi: 10.1038/ncomms3997 (2014).